Reply to ‘Sulfisoxazole does not inhibit the secretion of small extracellular vesicles’ 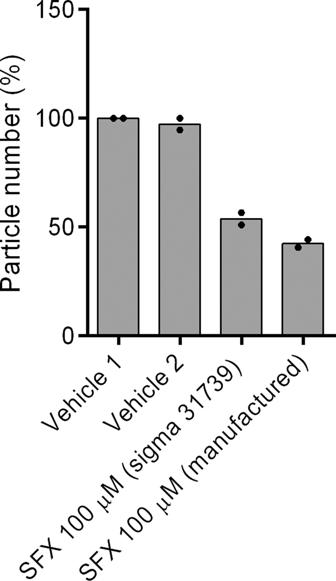Fig. 1: sEV secretion from MDA-MB-231 cells with or without SFX 100 µM (Sigma 31739, and manufactured SFX). All experiments were performed with a blind test (n= 2 biologically independent samples). Cells and cell culture MDA-MB231 cells were obtained from the American Type Culture Collection and grown at 37 °C under a humidified atmosphere with 5% CO 2 and 95% air using DMEM (Hyclone) with 10% FBS (Hyclone) and 1% antibiotic–antimycotic solution (AA, Hyclone). All cell lines were tested for mycoplasma contamination by polymerase chain reaction genotyping. Drugs SFX (31739) was purchased from Sigma-Aldrich. Manufactured SFX was synthesized and provided by Daegu-Gyeongbuk Medical Innovation Foundation, Republic of Korea. Isolation of sEVs and analysis Step 1 : Seed the 5 × 10 6 cells in 150-mm plate (20 ml DMEM with 10% FBS, 1% AA). Step 2 : After 24 h, wash using phosphate-buffered saline (PBS) and then change the media (20 ml DMEM without FBS, AA) with the drug. Step 3 : After 24 h, collect the cell culture supernatant. Step 4 : Centrifuge at 300 × g , 4 °C, 3 min and transfer the supernatants to a new tube. Step 5 : Centrifuge at 2500 × g , 4 °C, 20 min and transfer the supernatants to a new tube. Step 6 : Centrifuge at 10,000 × g , 4 °C, 30 min and transfer the supernatants to a new tube. Step 7 : Filter the supernatants using 0.22-µm syringe filters and transfer the supernatants to a new tube (#344058, Beckman Open-Top Tube). Step 8: Ultracentrifuge at 120,000 × g , 4 °C, 90 min. Step 9 : Resuspend sEV pellets with 30 ml PBS and centrifuge at 120,000 × g , 4 °C, 90 min again. Step 10 : Remove the supernatants and add the 1 ml PBS. Step 11 : After sealing the tube with parafilm, store at 4 °C, 1 h and resuspend the pellet. Step 12 : Transfer the samples to e-tube and analyze using NanoSight and GraphPad Prism. Reporting summary Further information on research design is available in the Nature Research Reporting Summary linked to this article.